Structural basis for trypanosomal haem acquisition and susceptibility to the host innate immune system Sleeping sickness is caused by trypanosome parasites, which infect humans and livestock in Sub-Saharan Africa. Haem is an important growth factor for the parasites and is acquired from the host by receptor-mediated uptake of haptoglobin (Hp)–haemoglobin (Hb) complexes. The parasite Hp–Hb receptor (HpHbR) is also a target for a specialized innate immune defence executed by trypanosome-killing lipoprotein particles containing an Hp-related protein in complex with Hb. Here we report the structure of the multimeric complex between human Hp–Hb and Trypanosoma brucei brucei HpHbR. Two receptors forming kinked three-helical rods with small head regions bind to Hp and the β-subunits of Hb (βHb), with one receptor at each end of the dimeric Hp–Hb complex. The Hb β-subunit haem group directly associates with the receptors, which allows for sensing of haem-containing Hp–Hb. The HpHbR-binding region of Hp is conserved in Hp-related protein, indicating an identical recognition of Hp–Hb and trypanolytic particles by HpHbR in human plasma. Sleeping sickness is caused by infection of humans and livestock by various forms of Trypanosoma brucei ( T.b. ) parasites and is a major health and socio-economical problem in large areas of Sub-Saharan Africa [1] . The parasites are protozoan hemoflagellates transmitted by tsetse flies to the host blood where they proliferate. Evasion of the host immune system is achieved by antigenic variation, in which a coating of variable surface glycoproteins (VSGs) on the parasite surface is constantly changing within the population [2] , [3] . Trypanosomes are deficient in haem biosynthesis and require uptake of exogenous haem [4] . Haem acquisition is mediated by the haptoglobin (Hp)–haemoglobin (Hb) receptor (HpHbR) located in the flagellar pocket of the parasite [5] . The receptor recognizes and takes up the Hp–Hb complex formed in the host’s bloodstream when Hb is released from erythrocytes during haemolysis. The trypanosome parasites themselves are reported to possess haemolytic activity [6] . This allows the parasite to steal the haem groups from Hb for incorporation into its own haemoproteins [5] . HpHbR is a 37-kDa receptor [5] structurally related to the glycophosphatidylinositol (GPI)-anchored trypanosomal VSGs [7] and the glutamic acid/alanine-rich protein, GARP, which replaces the VSGs in the tsetse midgut [8] . On the other hand, HpHbR is completely different from the mammalian Hp–Hb receptor, CD163 [9] . Besides its role in haem acquisition, HpHbR is also a target for primate innate immunity against certain trypanosome species [10] . In humans this is achieved through the action of trypanolytic particles (TLF1 or TLF2) that contain the primate-specific apolipoprotein L1 and Hp-related protein (Hpr) [11] , [12] , [13] . Hpr is a gene duplication product highly homologous to Hp [14] . TLF1 particles enter the parasite via HpHbR-mediated uptake [15] . The uptake of TLF1 requires Hb, which interacts with Hpr to form an Hpr–Hb complex [16] . As HpHbR, in contrast to CD163, also recognizes Hpr–Hb [5] , the entire TLF1 particle is endocytosed by the parasite [17] . Subsequently, apolipoprotein L1 forms a pore in the lysosomal membrane leading to a lethal release of lysosomal content into the parasite cytosol [18] , [19] , [20] , [21] . The two human pathogenic subspecies Trypanosoma brucei rhodesiense ( T.b. rhodesiense ) and Trypanosoma brucei gambiense ( T.b. gambiense ) express resistance proteins counteracting apolipoprotein L1 activity enabling these parasite strains to evade the lethal action of TLF particles [22] , [23] , [24] , [25] . T.b. gambiense also exhibits low-level HpHbR expression [26] and harbours a L210S substitution in HpHbR, leading to reduced TLF1 uptake [7] , [27] , [28] . These defence mechanisms are not present in the widespread Trypanosoma brucei brucei ( T.b. brucei ) subspecies, which is highly infectious in many non-primate species that do not express Hpr and apolipoprotein L. To investigate the mechanism of trypanosomal haem acquisition by HpHbR and its role in human immunity, we have determined the structure of the T.b. brucei HpHbR in complex with human Hp–Hb. The structure reveals an unexpected haem-sensing mechanism of HpHbR that appears conserved in trypanosome species. Furthermore, we show that the Hp–Hb epitope recognized by HpHbR is identical in TLF-associated Hpr–Hb, which explains the inability of trypanosomes to distinguish between the beneficial Hp–Hb and the lethal TLF1 particle. Structure determination For structural and functional analysis of the Hp–Hb–HpHbR complex, we purified Hp and Hb from human blood, while HpHbR (residues 36–378) was expressed in the yeast Pichia pastoris . Initial crystallization trials of the complex were unsuccessful. 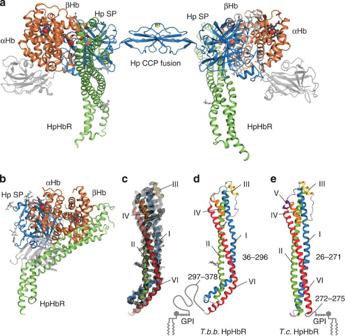Figure 1: Crystal structure of the Hp–Hb–HpHbR complex. (a) Cartoon representation of human Hp–Hb bound toT.b. bruceiHpHbR. Dimeric Hp is shown in blue, with complement control protein (CCP) domains forming a CCP fusion domain and the serine protease-like (SP) domain of Hp interacting with Hb and HpHbR. αHb and βHb are shown in orange and HpHbR in green. The haemoglobin-bindingStaphylococcus aureusIsdH NEAT1 domain (shown in transparent grey cartoons) was used as stabilizer in the crystallization process. Haem prosthetic groups are shown as dark-grey sticks with Fe atoms as red spheres. Glycosylations are shown as light-grey sticks and disulphide bridges as yellow sticks. (b) As inawith the view rotated by 90°. (c) Final 2mFo–DFc electron density map of one HpHbR receptor of the Hp–Hb–HpHbR crystal structure, displayed at 1.5σcontour level (black mesh). (d,e) Comparison ofT.b. bruceiHpHbR (d) andT. congolenseHpHbR (PDB code 4E40) (e). Helix I is coloured blue, helix II green, helix III yellow, helix IV orange, helix V purple and helix VI red. However, when the Hb-binding NEAT1 domain of Staphylococcus aureus IsdH was added to the complex, crystallization was achieved and data extending to 3.1 Å resolution were collected ( Table 1 ; Supplementary Fig. 1 ). The IsdH fragment appears to stabilize the complex and promote crystal formation by introducing crystal contacts ( Supplementary Fig. 2 ). IsdH NEAT1 interacts exclusively with the α-subunit of Hb (αHb) and is located distal to the receptor interface. Table 1 Data collection of refinement statistics. Full size table Structure of the Hp–Hb–HpHbR complex Hp (isoform 1) is a bivalent molecule owing to the association of its complement control protein (CCP) domains [29] . Each Hp moiety forms a tight interaction with an αβHb-dimer via its serine protease-like (SP) domain and the Hp–Hb complex has a barbell-like structure with αβHb loaded at the ends [30] , [31] . Our structure reveals that the dimeric Hp–Hb is recognized by two HpHbR receptors interacting with both the Hp SP domains and the β-subunits of Hb ( Fig. 1a,b ). The receptors are oriented perpendicular to the longitudinal axis of the Hp–Hb dimer with the membrane-associated ends pointing in the same direction, showing that two receptors are capable of cross-linking the ligand on the surface of trypanosome parasites. This avidity effect is likely to substantially increase the functional affinity of the interaction. A model of trimeric Hp(isoform 2)–Hb [30] bound to HpHbR supports that higher multimers of Hp–Hb that are present in humans carrying the Hp2 gene can also bind multiple receptors on the parasite surface ( Supplementary Fig. 3 ). These multimers may have even higher functional affinity for the receptors. Figure 1: Crystal structure of the Hp–Hb–HpHbR complex. ( a ) Cartoon representation of human Hp–Hb bound to T.b. brucei HpHbR. Dimeric Hp is shown in blue, with complement control protein (CCP) domains forming a CCP fusion domain and the serine protease-like (SP) domain of Hp interacting with Hb and HpHbR. αHb and βHb are shown in orange and HpHbR in green. The haemoglobin-binding Staphylococcus aureus IsdH NEAT1 domain (shown in transparent grey cartoons) was used as stabilizer in the crystallization process. Haem prosthetic groups are shown as dark-grey sticks with Fe atoms as red spheres. Glycosylations are shown as light-grey sticks and disulphide bridges as yellow sticks. ( b ) As in a with the view rotated by 90°. ( c ) Final 2mFo–DFc electron density map of one HpHbR receptor of the Hp–Hb–HpHbR crystal structure, displayed at 1.5 σ contour level (black mesh). ( d , e ) Comparison of T.b. brucei HpHbR ( d ) and T. congolense HpHbR (PDB code 4E40) ( e ). Helix I is coloured blue, helix II green, helix III yellow, helix IV orange, helix V purple and helix VI red. Full size image HpHbR residues 36–296 adopt a rod-like structure with a length of 110 Å and approximate diameter of 15 Å ( Fig. 1c,d ). It is composed of three long helices (I, II and VI) with two small helices (III and IV) forming a bulging head region at the membrane-distal end. No electron density is observed for the C-terminal region (residues 297–378), which is linked to the membrane via a GPI anchor, indicating a flexible or disordered structure. A single disulphide bridge (Cys 49 –Cys 197 ) connects helices I and III and thereby provides stability to the head region. The structure of T.b. brucei HpHbR is highly similar to the recently described structure of T. congolense HpHbR [7] ( Fig. 1d ) and 202 Cα atoms can be superimposed with a r.m.s.d. of only 2.2 Å. However, the two structures differ in the conformation of the membrane-associated end. T.b. brucei HpHbR has a bent conformation due to kinking of helices I, II and VI, whereas T. congolense HpHbR has a straight conformation. Furthermore, the C-terminal extension ( T.b. brucei HpHbR residues 297–378) is substantially shorter in T. congolense HpHbR (residues 272–275) ( Fig. 1d,e ). The difference in length may correlate with difference in thickness of the VSG coat in T.b. brucei and T. congolense , allowing both receptors to extend above the VSGs for interaction with Hp–Hb [7] . Binding interfaces The Hp–Hb–HpHbR structure also for the first time reveals the structure of the human Hp–Hb complex that has previously failed to form high-resolution diffracting crystals [32] . The human Hp–Hb is essentially similar to the recently determined porcine Hp–Hb complex [30] with two CCP domains merging into a CCP fusion domain via β-strand swapping ( Fig. 1a ). Hp–Hb binds along the side of HpHbR and interacts primarily with residues from helices I and II ( Fig. 2a ; Supplementary Fig. 4 ). The Hp-binding site on HpHbR is formed by residues from helix I (residues 68–85) and two residues from helix VI (residues 256 and 259), whereas the βHb-binding site is formed by residues from both helix I (residues 56–70) and helix II (residues 157–165) ( Fig. 2a ; Supplementary Fig. 4 ). Furthermore, residues from the loop region between helices III and IV (residues 200–202) also contact βHb. The interface between HpHbR and Hp buries a 1,618-Å 2 surface area, whereas the interface between HpHbR and βHb buries 1,491 Å 2 . In total, the interaction between Hp–Hb and HpHbR buries a 3,013-Å 2 surface area. 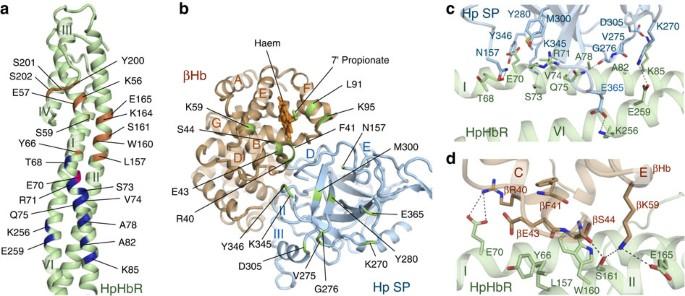Figure 2: Interactions between Hp–Hb and HpHbR. (a) Mapping of HpHbR residues interacting with Hp–Hb. Residues within 3.6 Å of Hp and Hb are coloured blue and orange, respectively. Glu70 is within 3.6 Å distance from both Hp and Hb and coloured magenta. (b) Hp and Hb residues within 3.6 Å distance from HpHbR are coloured green. Hp–Hb is related to HpHbR inaby a vertical rotation of 180°. Hb is shown in orange and Hp in light blue. Haem is shown as sticks. (c) Interactions between HpHbR (green) and Hp (blue). Dashed lines represent electrostatic interactions or hydrogen bonds. (d) Interactions between HpHbR (green) and Hb (orange). Figure 2: Interactions between Hp–Hb and HpHbR. ( a ) Mapping of HpHbR residues interacting with Hp–Hb. Residues within 3.6 Å of Hp and Hb are coloured blue and orange, respectively. Glu70 is within 3.6 Å distance from both Hp and Hb and coloured magenta. ( b ) Hp and Hb residues within 3.6 Å distance from HpHbR are coloured green. Hp–Hb is related to HpHbR in a by a vertical rotation of 180°. Hb is shown in orange and Hp in light blue. Haem is shown as sticks. ( c ) Interactions between HpHbR (green) and Hp (blue). Dashed lines represent electrostatic interactions or hydrogen bonds. ( d ) Interactions between HpHbR (green) and Hb (orange). Full size image Several surface-exposed loops from Hp are involved in binding to HpHbR. These are exclusively located in the second β-barrel subdomain of the serine protease-like domain, except for a single residue in the C-terminal part of the Hp α-chain (Asn157). In addition to van der Waals contacts, electrostatic interactions are formed between Hp Lys270 and HpHbR Glu259, Hp Asp305 and HpHbR Lys85 and Hp Glu365 and HpHbR Lys256 ( Fig. 2c ; Supplementary Fig. 4 ). Hydrogen bonds are formed between Hp Asn157 and the main chain carbonyl of Thr68 and between Hp Lys345 and HpHbR Ser73. Also, the main chain carbonyl of Gly276 forms a hydrogen bond with HpHbR Gln75. HpHbR recognizes residues from βHb helices C, E and F. From βHb helix C, Arg40 engages in electrostatic interactions with HpHbR Glu70 ( Fig. 2d ; Supplementary Fig. 4 ), whereas the main chain carbonyl of C-helix residue Ser44 forms a hydrogen bond with HpHbR Ser161. Lys59 from βHb helix C forms electrostatic interactions with HpHbR Glu165 and a hydrogen bond with HpHbR Ser161. From βHb F-helix, Lys95 form electrostatic interactions with HpHbR Glu57 and a hydrogen bond with the main chain carbonyl of HpHbR Ser202 ( Fig. 3a ; Supplementary Fig. 4 ). 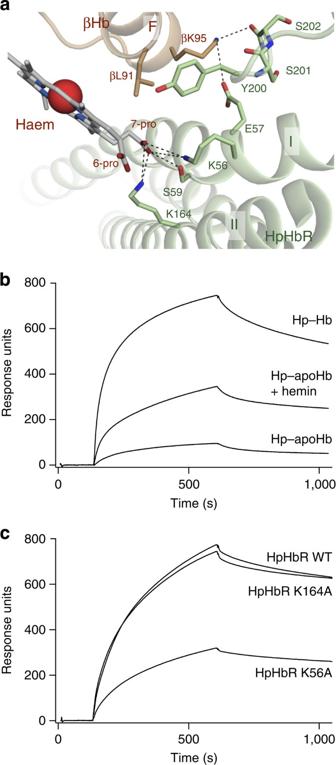Figure 3: Specific recognition of the βHb haem group is important for receptor–ligand interaction. (a) Interactions between HpHbR (green) and βHb/βHb haem group (grey sticks). Dashed lines represent electrostatic interactions or hydrogen bonds. (b) Surface plasmon resonance (SPR) analysis of Hp–Hb, Hp–apoHb and Hp–apoHb+hemin binding to immobilized HpHbR. (c) SPR analysis of HpHbR WT, K56A and K164A binding to immobilized Hp–Hb. Figure 3: Specific recognition of the βHb haem group is important for receptor–ligand interaction. ( a ) Interactions between HpHbR (green) and βHb/βHb haem group (grey sticks). Dashed lines represent electrostatic interactions or hydrogen bonds. ( b ) Surface plasmon resonance (SPR) analysis of Hp–Hb, Hp–apoHb and Hp–apoHb+hemin binding to immobilized HpHbR. ( c ) SPR analysis of HpHbR WT, K56A and K164A binding to immobilized Hp–Hb. Full size image Haem-sensing mechanism of HpHbR HpHbR specifically recognizes the βHb haem prosthetic group via electrostatic interactions between the two basic HpHbR residues Lys56 and Lys164 and the 7-propionate side chain of the haem group ( Fig. 3a ; Supplementary Fig. 5 ). HpHbR Lys164 coordinates the carboxylate of the haem 7-propionate side chain with a distance of 2.9 Å, whereas the distance between Lys56 and the carboxylate is 3.5 Å. To test the significance of the HpHbR recognition of the βHb haem group, we prepared samples of apoHb (without haem) by acid acetone precipitation of native human Hb ( Supplementary Fig. 6 ). Similar to native haem-containing Hb, apoHb forms a stable complex with Hp. Using surface plasmon resonance (SPR) with immobilized HpHbR, we show that Hp–apoHb binding to HpHbR is significantly reduced compared with native Hp–Hb ( Fig. 3b ). However, when hemin is added to Hp–apoHb the binding to HpHbR is partly restored. These results indicate that the interaction between the haem 7-propionate side chain and HpHbR is important for ligand binding. To further test this hypothesis, we mutated HpHbR residues Lys56 and Lys164 that interact directly with the 7-propionate side chain. The HpHbR K164A mutation shows the same binding properties to immobilized Hp–Hb as wild-type HpHbR, whereas the K56A mutation significantly reduces Hp–Hb affinity ( Fig. 3c ). These results show that both presence of haem on Hb and HpHbR Lys56 are important for the interaction between Hp–Hb and HpHbR, suggesting that direct recognition of the βHb haem group may be of functional importance for haem acquisition by trypanosome parasites. Although Lys164 is located closer to the haem 7-propionate side chain than Lys56 and may engage in a stronger interaction, our results show that it is not important for the interaction between Hp–Hb and HpHbR. HpHbR Ser59 possibly forms a hydrogen bond with the haem 7-propionate side chain, however, its electron density is not well defined suggesting a flexible conformation ( Supplementary Fig. 5 ). Furthermore, the HpHbR S59A mutant shows no decrease in Hp–Hb affinity ( Supplementary Fig. 7 ), indicating no functional significance of Ser59. Reduced Hp–Hb affinity of T.b. gambiense HpHbR A single amino-acid difference in T.b. gambiense HpHbR (Ser210) compared with T.b. brucei HpHbR (Leu210) leads to reduced affinity for human Hp–Hb and Hpr–Hb [7] , [27] , [28] . In combination with low-level expression of HpHbR [26] and the protective effect of TgsGP [22] , this evolutionary amino-acid substitution contributes to T.b. gambiense resistance against the human TLF particles. In T.b. brucei, Leu210 is positioned in HpHbR helix IV and its side chain is packed in the hydrophobic core of the head region ( Fig. 4 ). Substitution of leucine to serine at this position probably leads to an overall destabilization of the head region. In addition, HpHbR Leu210 is located only 8 Å from Lys56. Hence the L210S substitution may directly affect the structural properties of Lys56 and consequently the interaction with Hp–Hb and Hpr–Hb associated with TLF particles. 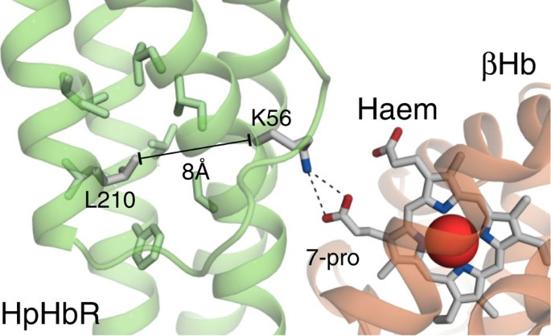Figure 4: L210S substitution inT.b. gambienselowers affinity for Hp–Hb. Position of Leu210 (Ser210 inTrypanosoma brucei gambiense) in the head region of HpHbR. Leu210 is located in a hydrophobic environment and its substitution to a hydrophilic serine may affect both the general stability of the head region and the position of Lys56, which is located only 8 Å away. Figure 4: L210S substitution in T.b. gambiense lowers affinity for Hp–Hb. Position of Leu210 (Ser210 in Trypanosoma brucei gambiense ) in the head region of HpHbR. Leu210 is located in a hydrophobic environment and its substitution to a hydrophilic serine may affect both the general stability of the head region and the position of Lys56, which is located only 8 Å away. Full size image Trypanosome parasites are experts in host immune system avoidance due to the VSGs that cover their surface. Only one form of VSG is expressed at a time, but the VGSs are constantly changing within the parasite population by means of gene conversion [3] , allowing the parasite to escape the adaptive immune system of the host. The VSGs forms an ~150-Å-thick tightly packed monolayer that prevents immunoglobulin recognition of epitopes embedded in the layer [33] , [34] , [35] . To bind and endocytose Hp–Hb or TLF particles, it has been suggested that HpHbR extends above the VSG layer [7] . In this paper, we present the structure of T.b. brucei HpHbR in complex with Hp–Hb, showing the exact binding site of Hp–Hb along the side of HpHbR. The Hp–Hb-binding site is located ~55 Å from the C-terminal end of HpHbR helix VI, which is connected to the membrane via an 82 amino-acid linker and a GPI anchor. We do not observe any electron density for this C-terminal linker region, probably because it is highly flexible. For the Hp–Hb-binding site to be presented above the VSG layer, the C-terminal linker region must span a distance of >95 Å. Considering the large number of amino acids constituting the linker, a length of 95 Å is achievable. With a ligand-binding region protruding from the VSGs a large part of HpHbR will be accessible from the host’s bloodstream and make the parasite susceptible to immunoglobulin attack. However, restricted access to the flagellar pocket where HpHbR is located and rapid endocytosis followed by antibody degradation may protect the parasite. Our structural analysis identified an unexpected interaction between HpHbR and the prosthetic haem group bound to βHb. Two HpHbR lysine residues Lys56 and Lys164 both engage in electrostatic interactions with the 7-propionate side chain of βHb haem. Affinity quantification by SPR analysis showed that mutation of Lys56 and removal of haem from Hb had a significant effect on binding, while mutation of Lys164 had no effect. On the basis of these results, we propose that HpHbR Lys56 serves as a haem sensor that enables HpHbR to discriminate between haem-associated Hp–Hb complexes and the corresponding apoprotein. Sequence conservation in an alignment of HpHbR from T. vivax , T. congolense and T.b. brucei mapped on the surface of HpHbR, shows moderate conservation among the three species ( Fig. 5a ; Supplementary Fig. 8 ). This includes the Hp–Hb-binding interface. However, the three residues Ser59, Lys164 and Asp168 are strictly conserved within the three species, whereas Lys56 is replaced by an alanine in T. congolense HpHbR or a serine in T. vivax HpHbR. Thus, the important role of T.b. brucei HpHbR Lys56 in ligand recognition is not conserved among trypanosome species. In T. congolense , HpHbR residues Ser59, Lys164 and Asp168 (Ser52, Lys153 and Asp157 in T. congolense HpHbR) are all essential for interaction with HpHbR [7] . Hence, it appears that the haem-sensing function of Lys56 may have shifted to Lys164 in T. congolense and T. vivax HpHbR. The essential roles of Ser59 and Asp168 in T. congolense HpHbR can be explained by their coordination of Lys164, which may stabilize the position of Lys164 and promote its interaction with the haem 7-propionate side chain ( Fig. 5b ). T.b. brucei HpHbR Ser59 coordinate Lys56 indicating a similar function of Ser59 in T.b. brucei and T. congolense . However, this is contradicted by our data showing that the S59A mutation in T.b. brucei HpHbR does not decrease its affinity for Hp–Hb. The specific role of T.b. brucei Asp168 in Hp–Hb binding could not be analysed, as the D168A mutant renders the protein unstable. 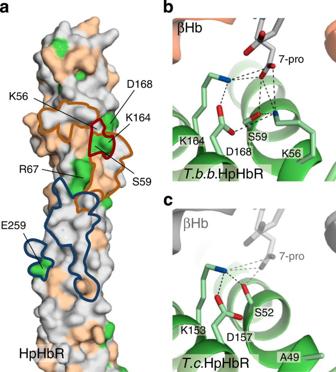Figure 5: Sequence variation in trypanosome species. (a) Sequence conservation in an alignment ofTrypanosoma brucei bruceiHpHbR,Trypanosoma congolenseHpHbR andTrypanosoma vivaxHpHbR is mapped on the surface ofT.b. bruceiHpHbR. Strictly conserved residues are coloured green and partly conserved residues are coloured beige and non-conserved residues are coloured grey. Blue outline indicates the Hp-binding interface, orange outline the Hb-binding interface and the red outline indicates residues that interact with the βHb haem group. (b,c) Comparison of βHb haem interaction sites inT.b. bruceiHpHbR (b) andT. congolenseHpHbR (c). InT. congolenseHpHbR, the positions of βHb and haem group (shown in grey) are modelled from the structure ofT.b. bruceiHp.Hb–HpHbR–IsdH NEAT1. Figure 5: Sequence variation in trypanosome species. ( a ) Sequence conservation in an alignment of Trypanosoma brucei brucei HpHbR, Trypanosoma congolense HpHbR and Trypanosoma vivax HpHbR is mapped on the surface of T.b. brucei HpHbR. Strictly conserved residues are coloured green and partly conserved residues are coloured beige and non-conserved residues are coloured grey. Blue outline indicates the Hp-binding interface, orange outline the Hb-binding interface and the red outline indicates residues that interact with the βHb haem group. ( b , c ) Comparison of βHb haem interaction sites in T.b. brucei HpHbR ( b ) and T. congolense HpHbR ( c ). In T. congolense HpHbR, the positions of βHb and haem group (shown in grey) are modelled from the structure of T.b. brucei Hp.Hb–HpHbR–IsdH NEAT1. Full size image To our knowledge, HpHbR is the first identified endocytic receptor that directly senses the presence of a prosthetic group within a carrier protein. Other endocytic receptors are able to detect prosthetic groups bound to their ligands, but in an indirect way. The mammalian endocytic receptor cubam that via its cubilin subunit is responsible for intestinal uptake of vitamin B 12 , a metal-binding haem-like tetrapyrrole, only recognizes the carrier protein, intrinsic factor, when it is in complex with vitamin B 12 (ref. 36 ). In this case vitamin B 12 indirectly promotes interaction with cubilin by locking the intrinsic factor in a specific conformation that allows a dual-point interaction with cubilin [37] . HpHbR is, as mentioned, also targeted by the human innate immune system via Hpr, which is incorporated in the trypanosome-killing TLFs. The gene encoding Hpr has arisen by a duplication of the Hp gene in primate evolution [38] . The Hpr amino-acid sequence is 91% identical to Hp, and the two proteins are predicted to have nearly identical three-dimensional structures [30] . Despite their structural similarity and common ability to bind Hb, Hp and Hpr serve quite different biological functions. Hp is responsible for binding and neutralizing the toxic Hb released from red blood cells and subsequent scavenging by macrophages via its interaction with the receptor CD163 (refs 9 , 39 ), whereas Hpr in complex with Hb mediates delivery of toxic TLF particles to trypanosome parasites [16] , [17] . Our data reveal, in atomic detail, the interaction between Hp and HpHbR, and an alignment of Hp and Hpr shows that residues interacting with HpHbR are conserved ( Fig. 6a ; Supplementary Fig. 9 ). Therefore, Hp–Hb and Hpr–Hb most likely form identical interactions with HpHbR, and the structure of the Hp–Hb–HpHbR complex therefore applies to both the haem acquisition mechanism and the human innate immunity against trypanosome parasites ( Fig. 6b ). As the structural epitopes presented to the parasites by Hp–Hb and Hpr–Hb contained in TLF particles are identical, the parasites are incapable of distinguishing between the beneficial Hp–Hb complex and the lethal TLF particles. On the other hand, the Hp interface with HpHbR is completely distinct from the Hp region known to interact with the mammalian Hp–Hb receptor, CD163 ( Fig. 6a ). The interaction with CD163 involves two basic Hp-specific residues (Arg311 and Lys321) located in the loop 3 region [40] . These residues engage in a common type electrostatic and calcium-dependent binding to the scavenger receptor cysteine-rich domains of CD163 (refs 41 , 42 ). These two essential basic residues are not present in Hpr and consequently Hpr–Hb is not recognized by CD163 (ref. 41 ). This prevents an unfavourable CD163-mediated clearance of TLFs from circulation, while HpHbR-mediated uptake of TLF1 by infecting trypanosome parasites is maintained. 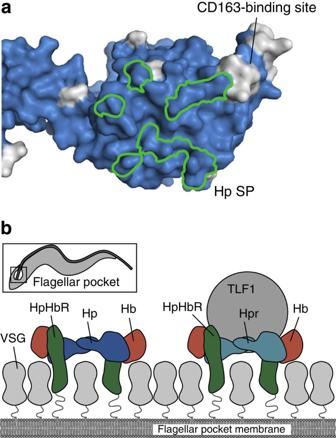Figure 6: Hp–Hb/TLF1 uptake by HpHbR. (a) Sequence conservation in an alignment of human Hp and Hpr mapped on the surface of Hp. Conserved residues are coloured blue and non-conserved residues grey. Green outline indicates the HpHbR-binding site. (b) Schematic drawing of HpHbR involvement in nutritional uptake of Hp–Hb (left) and susceptibility to the human immune system via uptake of Hpr–Hb associated to TLF1 particles (right). HpHbR is expressed exclusively in the flagellar pocket of the parasite5as indicated by the black box. Figure 6: Hp–Hb/TLF1 uptake by HpHbR. ( a ) Sequence conservation in an alignment of human Hp and Hpr mapped on the surface of Hp. Conserved residues are coloured blue and non-conserved residues grey. Green outline indicates the HpHbR-binding site. ( b ) Schematic drawing of HpHbR involvement in nutritional uptake of Hp–Hb (left) and susceptibility to the human immune system via uptake of Hpr–Hb associated to TLF1 particles (right). HpHbR is expressed exclusively in the flagellar pocket of the parasite [5] as indicated by the black box. Full size image Treatment of human sleeping sickness caused by T.b. gambiense and T.b. rhodesiense is currently restricted to drugs developed over four decades ago [43] , [44] . Although efficacious in some cases, these drugs are far from ideal due to the complexity in their medical administration as well as emerging resistance. Consequently, the development of new medical treatments is needed. The new insight into the molecular ligand recognition by the HpHbR may provide a framework for design of compounds that target HpHbR. One tempting approach is to exploit HpHbR for delivery of toxic and parasite-killing compounds to the parasite. Another approach is to design compounds that inhibit HpHbR-medidated Hp–Hb uptake and thereby restrict parasite haem acquisition and growth. Purification of Hp–Hb from human blood Anti-coagulant (trisodium citrate and EDTA) was added to human blood (from a homozygotic Hp1 donor) to a final concentration of 15 mM (trisodium citrate) and 0.15 mM (EDTA). Plasma and blood cells were separated by centrifugation at 4,000 g for 20 min. The blood cell fraction was lysed by addition of water (1:1 ratio) and cell debris was removed by centrifugation at 8,000 g for 15 min. Clotting factors were removed from plasma by addition of 80 mM BaCl 2 , followed by incubation on ice for 1 h and centrifugation at 27,000 g for 15 min. Serum and blood cell fractions were stored at −80 °C. Thawed serum and blood cell fractions were mixed in a ratio of 25:1 and incubated at 4 °C overnight. The sample was diluted 1:2 in 20 mM Tris–HCl pH 7.6 and loaded on a Blue Sepharose Fast Flow column (GE healthcare) equilibrated in 50 mM KCl, 20 mM Tris–HCl pH 7.6. The flow-through was collected and loaded on a Q Sepharose Fast Flow column (GE Healthcare) equilibrated with buffer Q-A (50 mM KCl, 20 mM Tris–HCl pH 7.6). A gradient from 10 to 70% buffer Q-B (500 mM KCl, 20 mM Tris–HCl pH 7.6) was applied. Fractions containing Hp–Hb were pooled and ammonium sulphate added to 55% saturation. The sample was centrifuged at 27,000 g for 15 min and loaded on a Source 15 Iso column (GE Healthcare) equilibrated with buffer Iso-A (55% ammonium sulphate, 20 mM Tris–HCl, pH 7.6). A gradient from 0 to 100% buffer Iso-B (20 mM Tris pH 7.6) was applied. Fractions containing Hp–Hb were pooled and concentrated using an Amicon Ultra centrifugal filter (10 kDa molecular mass cut-off (MWCO), Millipore). The sample was further purified using a Superdex 200 column (GE Healthcare) equilibrated in 75 mM KCl, 20 mM Tris–HCl pH 7.6. Fractions containing Hp–Hb were pooled and concentrated to 2 mg ml −1 using an Amicon Ultra centrifugal filter (10 kDa MWCO, Millipore). Expression and purification of HpHbR wild type and mutants The gene encoding the trypanosoma brucei brucei HpHbR (residues 36–378) was amplified (primer: 5′-CCCACGAATTCGCTGAGGGTTTAAAAACCAAAGACGAAGTTG-3′, primer: 5′-GATTTGCGGCCGCTTAACTAACCACGTCAACGGGCCTTGG-3′) and cloned into the EcoRI and NotI sites of the pPICZαA vector and transformed into the P. pastoris X33 cell line (Life technologies). Point mutations were introduced in the vector using the site-directed, ligase-independent mutagenesis method [45] . Colonies expressing recombinant HpHbR were inoculated in buffered glycerol-complex medium and incubated at 30 °C for 24 h. Cells were transferred to buffered methanol-complex medium and grown for 72 h at 30 °C. Protein expression was induced by adding 1.5% methanol every 12 h. Secreted HpHbR was purified from the medium by diluting 1:5 with 20 mM Tris–HCl pH 7.6 and loading on a Q Sepharose Fast Flow column (GE Healthcare) equilibrated in buffer Q-A (50 mM KCl, 20 mM Tris–HCl, pH 7.6). A gradient from 15 to 80% buffer Q-B (500 mM KCl, 20 mM Tris–HCl pH 7.6) was applied. Fractions containing HpHbR were pooled and concentrated using an Amicon Ultra centrifugal filter (10 kDa MWCO, Millipore). The sample was further purified using a Superdex 200 column (GE Healthcare) equilibrated in 75 mM KCl, 20 mM Tris–HCl, pH 7.6. HpHbR was deglycosylated by addition of 1/10 (w/w) endoglycosidase H and incubation overnight at 25 °C. Expression and purification of IsdH NEAT1 The gene encoding IsdH NEAT1 (residues 86–229) with an N-terminal His-tag followed by a thrombin cleavage site was synthesized and cloned into the NdeI and BamHI sites of the pET-22b(+) vector (Genscript, Novagen). The vector was transformed into the BL21 rosetta Escherichia coli strain. Protein expression was induced with 1 mM IPTG. Cells were harvested and resuspended in lysis buffer (500 mM KCl, 20 mM Tris–HCl pH 7.6, 20 mM imidazole, 1 tablet Complete protease inhibitor (Roche Diagnostics GmBH) and 10% glycerol). The cells were opened by sonication (Branson Sonifier 250) and centrifuged 27,000 g for 20 min. Prior to loading on a Ni-column the samples were filtered through a 0.22-μm filter. The protein was eluted from the Ni-column with a gradient from 20–300 mM imidazole in a buffer containing 20 mM Tris–HCl pH 7.6, 500 mM KCl and 10% glycerol. Fractions containing IsdH were pooled and dialysed overnight against 75 mM KCl, 20 mM Tris–HCl pH 7.6 and 10% glycerol. The His-tag was removed by addition of 1/100 (w/w) thrombin and incubation overnight at 25 °C. Formation and purification of the Hp–Hb–HpHbR–IsdH complex Hp–Hb, HpHbR and IsdH NEAT1 were mixed in 1:2:2 molar ratios and incubated overnight at 4 °C. The sample was loaded on to a Superdex 200 column (GE healthcare) equilibrated in 75 mM KCl, 20 mM Tris–HCl, pH 7.6. Fractions containing the Hp–Hb–HpHbR–IsdH NEAT1 complex were pooled and concentrated to 10 mg ml −1 using an Amicon Ultra centrifugal filter (10 kDa MWCO, Millipore). Crystallization and data collection Crystals were obtained at 4 °C using the sitting-drop vapour diffusion method. Two μl protein sample (10 mg ml −1 ) was mixed with 2 μl reservoir solution containing 15% polyethylene glycol 1500 and 0.1 M Bis-Tris pH 6.0. The crystals were transferred to the cryoprotection buffer (40% polyethylene glycol 1500 and 0.1 M Bis-Tris pH 6.0) before being flash frozen in liquid nitrogen. X-ray diffraction data were collected at the XO6SA beamline (Swiss Light Source, Villigen, Switzerland) using a wavelength of 1.0 Å and at a temperature of 100 K. Data were indexed, integrated and scaled with the XDS package [46] . The crystals display P2 1 symmetry and diffract to a maximal resolution of 3.1 Å, However, the data are highly anisotropic with diffraction limit at ~4.5 Å on the c * axis [47] ( Table 1 ). The structure was solved by molecular replacement in PHASER [48] with porcine Hp–Hb [30] , Hb–IsdH NEAT1 [49] and T. congolense HpHbR [7] as search models. Each asymmetric unit contains three dimeric Hp–Hb–HpHbR–IsdH complexes. Model building was done in the programs ‘O’ [50] and ‘Coot’ [51] . Iterative refinement cycles were performed in PHENIX [52] . Atomic coordinates were restrained by tight sixfold non-crystallographic symmetry (one group for each monomeric unit of Hp–Hb–HpHbR–IsdH) with one B-factor group per residue throughout the refinement procedure. Figures were made using PYMOL [53] . Formation and purification of the Hp–apoHb complex Extraction of haem from Hb was achieved by acid-acetone precipitation [54] . Hb (5 mg ml −1 ) was slowly added to ice-cold acid acetone (5 ml of 5 M HCl per litre HPLC-grade acetone) in a 1:25 v/v ratio. After incubation for 1 h on ice, the sample was centrifuged at 25,000 g for 10 min. The pellet was resuspended in 0.1 M acetic acid and used for another round of precipitation. This was repeated until no more haem could be detected in the supernatant. At this point the precipitated apoHb was dissolved in buffer containing 150 mM NaCl, 4 mM CaCl 2 and 10 mM HEPES pH 7.6. The sample was subsequently dialysed overnight against the same buffer. ApoHb was mixed with Hp in a 1:2 molar ratio and the Hp–apoHb complex purified using a Superdex 200 column (GE healthcare) equilibrated in 75 mM KCl and 20 mM Tris–HCl, pH 7.6. HoloHb was reconstituted by addition of 20 × molar excess of hemin prior to gelfiltration. Detection of haem was done by SDS–polyacrylamide gel electrophoresis and subsequent staining for peroxidase activity [55] and by ultraviolet–vis absorption spectroscopy on a UltroSpec 3100 spectrophotometer (GE Healthcare). Surface plasmon resonance Binding studies were performed on a Biacore 3000 instrument (GE Healthcare GmbH). Immobilization was conducted in 10 mM sodium acetate pH 4.0 and remaining sites were blocked with 1 M ethanolamine pH 8.5. The signal generated for T.b. brucei HpHbR was 71.4 fmol mm −2 and 42.6 fmol mm −2 for Hp–Hb. Sample and flow buffer was 150 mM NaCl, 1.5 mM CaCl 2 , 1.0 mM EGTA, 0.005% Tween-20 and 10 mM HEPES pH 7.6. Sensor chips were regenerated with 500 mM NaCl, 20 mM EDTA and 10 mM glycine pH 4.0. Accession codes: Atomic coordinates and structure factors for the Hp–Hb–HpHbR–IsdH NEAT 1 complex have been deposited in the Protein Data Bank under accession code 4WJG. How to cite this article: Stødkilde, K. et al. Structural basis for trypanosomal haem acquisition and susceptibility to the host innate immune system. Nat. Commun. 5:5487 doi: 10.1038/ncomms6487 (2014).